Polarity of bacterial magnetotaxis is controlled by aerotaxis through a common sensory pathway Most motile bacteria navigate within gradients of external chemical stimuli by regulating the length of randomly oriented swimming episodes. Magnetotactic bacteria are characterized by chains of intracellular ferromagnetic nanoparticles and their ability to sense the geomagnetic field, which is believed to facilitate directed motion, but is not well understood at the behavioural and molecular level. Here, we show that cells of Magnetospirillum gryphiswaldense unexpectedly display swimming polarity that depends on aerotactic signal transduction through one of its four chemotaxis operons ( cheOp1 ). Growth of cells in magnetic fields superimposed on oxygen gradients results in a gradual inherited bias of swimming runs with one of the cell poles leading, such that the resulting overall swimming direction of entire populations can be reversed by changes in oxygen concentration. These findings clearly show that there is a direct molecular link between aerotactic sensing and the determination of magnetotactic polarity, through the sensory pathway, CheOp1. One of the most intriguing examples of magnetic navigation in living organisms is magnetotaxis exhibited by certain aquatic bacteria, which synthesize nano-sized intracellular ferrimagnetic crystals of magnetite (Fe 3 O 4 ) or greigite (Fe 3 O 4 ), enclosed in the membrane-enveloped magnetosomes [1] . The chain-like arrangement of magnetosome particles generates a magnetic dipole that passively rotates the bacterium into alignment with the ambient magnetic field ( B ) as it swims actively by means of flagella [1] . Magnetotaxis is assumed to reduce the biased three-dimensional swimming pattern shown by most motile bacteria to linear movement along the geomagnetic field lines, which is believed to facilitate navigation to growth-favouring zones close to the oxic–anoxic transition in chemically stratified aquatic environments [2] . However, the biological mechanisms governing magnetotaxis have remained poorly understood [3] . In the classical aerobic hanging drop assay, most naturally occurring magnetotactic bacteria (MTB) exhibit a uniform, polar swimming pattern (defined as swimming polarity), that is, they persistently migrate either parallel or antiparallel to B , which is equivalent to movement towards or away, respectively, from the magnetic south pole of a bar magnet (that is, the pole that attracts the North-pointing end of a magnetic compass needle). Migration parallel or antiparallel to B is called North-seeking (NS) or South-seeking (SS) swimming polarity, respectively. Swimming polarity (either NS or SS) of individual cells results from the m agnetic polarity (M polarity) of the magnetosome chain with respect to the c ellular polarity (C polarity) caused by some sort of cellular asymmetry such as, for instance, monopolar flagellation. In the original model of magnetotaxis only a small fraction of cells was assumed to reverse M polarity in each generation [4] and cells were suggested to display only unidirectional motion [5] . This seemed to be consistent with the predominance of NS and SS MTB collected from environments in the northern and southern hemisphere [2] , respectively, which would guide MTB downwards along the opposing inclinations of the geomagnetic field in the two hemispheres to reach their microhabitat at the bottom of natural waters. More recently it was shown, however, that monopolarly flagellated MTB such as Magnetococcus marinus MC-1 reverse their swimming direction to alternate between upper and lower oxygen threshold levels by an unknown mechanism [6] , [7] . In contrast, bipolarly flagellated magnetospirilla such as the alphaproteobacterium Magnetospirillum gryphiswaldense that seemingly lack C polarity [8] were assumed to employ ‘axial magnetotaxis’, as cells were observed to swim aligned with magnetic field lines, but to lack a clear swimming polarity [6] , [9] , [10] . M. gryphiswaldense has been widely used as a model in many recent studies on magnetosome biosynthesis [11] . However, there has been little investigation of its motility and taxis [8] , [12] , [13] , and it is currently not known whether or how the magnetic behaviour of M. gryphiswaldense and other MTB is integrated with other sensory responses at the behavioural and molecular level, or whether it uses a dedicated sensing and signalling machinery. Here, we studied in detail the motility and behavioural responses of M. gryphiswaldense to defined oxygen concentrations. We found that aerotaxis is the dominant sensory system controlling swimming reversals. Unexpectedly, swimming polarity can be selected by serial growth in oxygen gradients with superimposed parallel magnetic fields, and the cells’ predominant swimming direction with respect to B can be instantaneously reversed by sudden changes in oxygen concentration. Both aerotaxis (that is, control of reversal rate irrespective of (magnetic) directionality) and swimming polarity (that is, control of swimming directionality with respect to the magnetic field) depend on the chemotaxis proteins encoded in just one of the four chemotaxis operons of M. gryphiswaldense , suggesting a direct molecular link between both navigational mechanisms. Aerotaxis is the dominant tactic behaviour In spatial chemotaxis assays, we observed a strong microaerophilic (that is, both aerophilic and -phobic) response, which obscured any other putative tactic reactions tested (for example, to light or carbon sources, see Methods for details). Cells accumulated as sharp bands within oxygen gradients ( Fig. 1a,b ). In the absence of oxygen, cells developed distinct tactic bands at millimolar concentrations in gradients of nitrate (an alternative terminal electron acceptor for anaerobic respiration [14] , Supplementary Fig. 1a ), indicating that the strong aerotaxis behaviour is part of a general energy taxis response similar to that identified in the microaerophilic A. brasiliense and other bacteria [15] , [16] , [17] , [18] . Swimming speeds of bacteria in the dense cell suspensions under a coverslip (uncontrolled oxic conditions) ranged between 20 and 60 μm s −1 ( Fig. 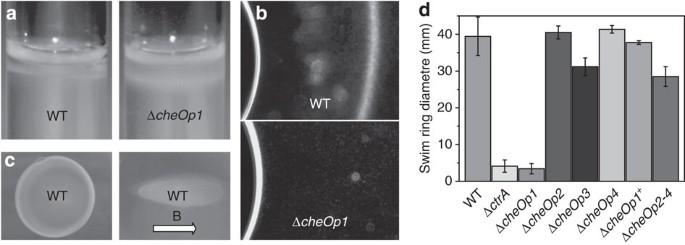Figure 1: Aerotactic behaviour ofM. gryphiswaldense. (a) Band formation of WT (left) and ΔcheOp1mutant (right) cells in soft agar tubes 2 days after inoculation. Unlike the sharp band observed for the WT, ΔcheOp1grew as a diffuse zone more distant to the agar surface. (b) Aerotactic band formation in a flat capillary 5 min after filling. (c) Swim ring formation of WT in 0.2% motility agar in the absence and presence of magnetic field (B). Orientation ofBis indicated (black arrow). (d) Swim ring formation of WT and mutant strains in 0.2% motility agar 2 days after inoculation (mean±s.d. of three independent replicates). Deletion ofcheOp1reduced swim ring size to the level of a non-motile ΔctrAmutant, which lacks any flagella filaments similar as described previously56.Cis-complementation of the ΔcheOp1mutant strain (ΔcheOp1+) restored WT-like behaviour. 2c ) with a mean of 41.6±3.5 μm s −1 ( Supplementary Table 1 ). Typically, bacteria exhibited long unidirectional runs of over several hundred micrometres ( Fig. 2a,b and Supplementary Movie 1 ), interrupted by short (<150 ms) reversal events (mean frequency 0.031±0.007 s −1 ). About 50% of cells that tethered spontaneously to the cover slip by one of their two bipolar flagella rotated unidirectionally either CW or CCW for at least 1 min ( Fig. 2d , Supplementary Movie 2 ), while the others reversed rotation at rates of up to 0.45 s −1 , suggesting reversals are caused, as in other bacteria, by reversal of the direction of motor rotation. Figure 1: Aerotactic behaviour of M. gryphiswaldense . ( a ) Band formation of WT (left) and Δ cheOp1 mutant (right) cells in soft agar tubes 2 days after inoculation. Unlike the sharp band observed for the WT, Δ cheOp1 grew as a diffuse zone more distant to the agar surface. ( b ) Aerotactic band formation in a flat capillary 5 min after filling. ( c ) Swim ring formation of WT in 0.2% motility agar in the absence and presence of magnetic field ( B ). Orientation of B is indicated (black arrow). ( d ) Swim ring formation of WT and mutant strains in 0.2% motility agar 2 days after inoculation (mean±s.d. of three independent replicates). Deletion of cheOp1 reduced swim ring size to the level of a non-motile Δ ctrA mutant, which lacks any flagella filaments similar as described previously [56] . Cis -complementation of the Δ cheOp1 mutant strain (Δ cheOp1 + ) restored WT-like behaviour. 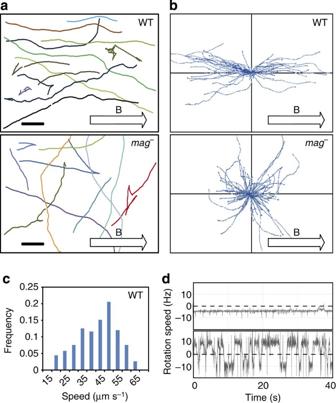Figure 2: Run and reversal motility behaviour ofM. gryphiswaldense. (a) Representative tracks of WT and non-magnetic ΔmamABmutant cells under a coverslip exposed to air in a homogenous horizontal magnetic field of 0.26 mT (B; orientation indicated by arrow). The bar represents 100 μm. (b) Plot of all recorded tracks of WT and non-magnetic ΔmamABmutant cells in a standard wet mount in a homogenous horizontal magnetic field of 0.26 mT (B). (c) Histogram depicting frequency versus swimming speed of WT cells in a standard wet mount. (d) Rotation diagrams of representative tethered WT cells. An extreme case of a cell rotating exclusively CCW (top) and a reversing cell (bottom) is shown. Movies were recorded at 43 fps and analysed using BRAS software57. Full size image Figure 2: Run and reversal motility behaviour of M. gryphiswaldense . ( a ) Representative tracks of WT and non-magnetic Δ mamAB mutant cells under a coverslip exposed to air in a homogenous horizontal magnetic field of 0.26 mT ( B ; orientation indicated by arrow). The bar represents 100 μm. ( b ) Plot of all recorded tracks of WT and non-magnetic Δ mamAB mutant cells in a standard wet mount in a homogenous horizontal magnetic field of 0.26 mT ( B ). ( c ) Histogram depicting frequency versus swimming speed of WT cells in a standard wet mount. ( d ) Rotation diagrams of representative tethered WT cells. An extreme case of a cell rotating exclusively CCW (top) and a reversing cell (bottom) is shown. Movies were recorded at 43 fps and analysed using BRAS software [57] . Full size image We studied the swimming responses of individual bacteria to defined oxygen concentrations at low cell densities within a microscopic gas perfusion chamber ( Supplementary Fig. 2 ) by employing automated video tracking. To separate the effects of magnetic fields from aerotactic behaviour, we first analysed an isogenic non-magnetic ( mag − ) Δ mamAB mutant [19] , whose swimming speed and reversal frequency were virtually undistinguishable from the magnetic WT ( Supplementary Table 1 , Supplementary Fig. 3d , Supplementary Movie 3 ). At a concentration of 1% and 5% oxygen, the mean speed of Δ mamAB was 4–7 μm s −1 higher than under anoxic conditions (33.3±10.6 μm s −1 ) ( Supplementary Fig. 3a ). Conversely, reversal rates were the highest under anoxic conditions (0.126±0.051 s −1 ) and the lowest at 5% oxygen (0.055±0.010 s −1 ). 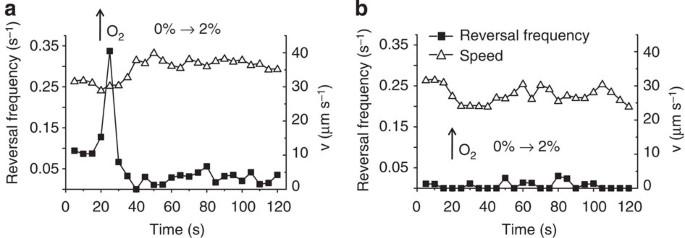Figure 3: Addition of oxygen triggers a distinct reversal response. Reversal rates and swimming speeds of ΔmamAB(a) and ΔcheOp1(b) cells recorded in the gas perfusion chamber subjected to an abrupt shift from 0 to 2% oxygen after 20 s (↑O2). Mean values of reversal frequency and speed of three independent experiments calculated for 5-s intervals are shown. On average 61 (a) and 17 (b) cells were tracked for each graph over the whole duration of the experiment. Abruptly shifting from micro-oxic (2% O 2 ) to anoxic conditions resulted in a slow but sustained decrease in swimming speed and in an increase in reversal frequency (approximately from 0.05 to 0.1 s −1 ) ( Supplementary Fig 3b ). A reverse shift (that is, challenging anoxic-adapted cells with 2% O 2 ) had a more pronounced effect and led to a transient threefold increase in reversal frequency ( Fig. 3a , Supplementary Movie 4 ). Within 5s post-shift, the prestimulus frequency of around 0.1 s −1 instantaneously increased to 0.34 s −1 . However, 10s post-shift this drastic response was followed by a drop in reversal frequency to below prestimulus levels, reaching nearly zero after 20 s. In contrast to other bacteria that rapidly adapt and return to prestimulus levels, in the following 80 s, the frequency remained low (average 0.03±0.02 s −1 ), resulting in long uninterrupted swimming runs. Figure 3: Addition of oxygen triggers a distinct reversal response. Reversal rates and swimming speeds of Δ mamAB ( a ) and Δ cheOp1 ( b ) cells recorded in the gas perfusion chamber subjected to an abrupt shift from 0 to 2% oxygen after 20 s (↑O 2 ). Mean values of reversal frequency and speed of three independent experiments calculated for 5-s intervals are shown. On average 61 ( a ) and 17 ( b ) cells were tracked for each graph over the whole duration of the experiment. Full size image Deletion of cheOp1 abolishes aerotaxis Analysis of the M. gryphiswaldense genome for genes that might encode proteins involved in aerotaxis revealed at least 56 genes encoding putative chemoreceptors [20] , known as m ethyl-accepting c hemotaxis p roteins (MCPs) ( Supplementary Table 3 ), and four putative chemotaxis operons designated cheOp1-4 ( Fig. 4 ). Highly conserved syntenic operons are also present in the related M. magneticum and M . magnetotacticum ( Supplementary Table 2 ). cheOp1 homologues belong to the well-conserved F5 class of chemotaxis systems [21] , so far almost exclusively found among alphaproteobacteria, whereas cheOp2 and cheOp3 homologues belong to the ACF class [21] . All operons encode the canonical set of chemotaxis genes cheA , cheW , cheY , cheB and cheR (although cheOp2 only has a hybrid cheY homologue) plus additional che homologues and putative chemotaxis-related genes encoding MCP, ParA-like [22] , EAL or GGDEF [23] domain proteins in cheOp2-4 . The best hits are to orthologues from other magnetotactic alphaproteobacteria ( Supplementary Table 2 ) followed by P. molischianum and different Rhodospirillum and Azospirillum species. Except for cheOp3 , representatives from all operons have been shown to be expressed [24] , [25] . 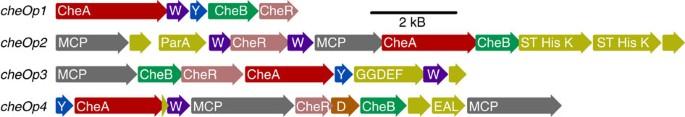Figure 4: Molecular organization of chemotaxis operons ofM. gryphiswaldense. Homologues of the same family are indicated by the same colour. W=cheW, Y=cheY, D=cheD, ST His K= signal transduction histidine kinase, GGDEF+EAL=genes encoding proteins containing the respective domains. Figure 4: Molecular organization of chemotaxis operons of M. gryphiswaldense . Homologues of the same family are indicated by the same colour. W= cheW , Y= cheY , D= cheD , ST His K= signal transduction histidine kinase, GGDEF+EAL=genes encoding proteins containing the respective domains. Full size image We constructed deletion mutants of all operons in the magnetic ( mag + ) WT background. Growth and magnetosome formation of all resulting mutant strains was not affected and motility was very similar to that of the WT, except that the average swimming speed of Δ cheOp1 was slightly reduced ( Fig. 3 ). Single deletions of cheOp2 , cheOp3 and cheOp4 had no detectable effect on aerotaxis, although Δ cheOp3 formed slightly smaller halos in swim agar plates ( Fig. 1d ). Halo size of a triple-deletion mutant, in which cheOp2-4 were eliminated successively, was the same as for Δ cheOp3, indicating that none of these operons is playing a major role in energy taxis. In striking contrast, deletion of cheOp1 caused a complete loss of the aerotactic response (= aer − ). Δ cheOp1 produced no tactic bands in either nitrate gradients ( Supplementary Fig. 1 ) or liquid medium in flat capillaries exposed to air ( Fig. 1b ), but grew as a diffuse zone close to the surface in soft agar oxygen gradients, unlike the sharp band observed for the WT ( Fig. 1a ). When Δ cheOp1 cells were subjected to an oxygen shift from 0 to 2%, they failed to display any behavioural changes, and, unlike the drastic response observed for the WT, reversal frequency remained around zero during the entire experiment ( Fig. 3b ), resulting in long, uninterrupted runs ( Supplementary Movie 5 ). The sensory pathway encoded by cheOp1 is therefore the only one controlling aerotaxis. Magnetic swimming polarity is controlled by aerotaxis In a magnetic field of 0.26 mT (about 5 × the strength of the geomagnetic field) the swimming tracks of WT ( mag + ) cells approximated to more or less straight lines ( Fig. 2a,b and Supplementary Movie 1 ). Distorted swimming halos reflecting the orientation of B were formed by the WT inoculated into motility agar exposed to magnetic fields ( Fig. 1c ). Swimming characteristics of Δ mamAB ( mag − ) cells were very similar to those of the WT, except that swimming paths were less straight and not magnetically aligned ( Supplementary Table 1 , Supplementary Movie 3 ). In the classical aerobic hanging drop assay ( Supplementary Fig. 4 ), WT cells grown under standard laboratory conditions (that is, in the absence of defined magnetic fields and at permanent agitation) accumulated in approximately equal numbers at both edges of the drop without detectable polarity ( pol − ), whereas Δ mamAB did not show any accumulation ( Fig. 5 and Supplementary Fig. 5g ). 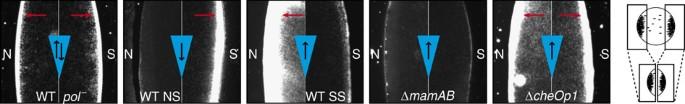Figure 5: Selection of magnetic swimming polarity depends on CheOp1. Dark field microsocopy images of WT and mutant cells at × 100 magnification in hanging drop assays exposed to air. Horizontal magnetic fields were applied with a permanent magnet and cells that accumulated at the drop edges corresponding to the north and south magnetic pole (indicated by N and S, respectively) were imaged. Both individual and densely packed cells are visible in dark field microscopy images as white dots or areas (accumulations highlighted by red arrows). For each representative sample, both edges of the same drop are shown (as illustrated in schematic (right)). Except for non-selected WT cells (pol−), all cultures were grown under selective conditions for at least two passages to select NS and SS cells. Orientation of the magnetic field (black arrows) with respect to the O2gradient (blue triangle) during selective growth is indicated. Figure 5: Selection of magnetic swimming polarity depends on CheOp1. Dark field microsocopy images of WT and mutant cells at × 100 magnification in hanging drop assays exposed to air. Horizontal magnetic fields were applied with a permanent magnet and cells that accumulated at the drop edges corresponding to the north and south magnetic pole (indicated by N and S, respectively) were imaged. Both individual and densely packed cells are visible in dark field microscopy images as white dots or areas (accumulations highlighted by red arrows). For each representative sample, both edges of the same drop are shown (as illustrated in schematic (right)). Except for non-selected WT cells ( pol − ), all cultures were grown under selective conditions for at least two passages to select NS and SS cells. Orientation of the magnetic field (black arrows) with respect to the O 2 gradient (blue triangle) during selective growth is indicated. Full size image The behaviour observed for non-selected cells was consistent with so-called ‘axial’ magnetotaxis. However, as previous observations indicated that magnetospirilla freshly isolated from environmental samples displayed strong swimming polarity [26] , [27] , we tested whether polarity could be reinduced in our M. gryphiswaldense WT lab strain [28] , which has been passaged for many generations in the absence of magnetic selection. We therefore performed serial transfers of cells in oxygen gradients (Ox Low →Ox High ), exposing them to either parallel (north pole→south pole) or antiparallel (south pole←north pole) magnetic fields of approximately 10 × the geomagnetic field strength (0.57 mT) (=selective conditions, Supplementary Fig. 4a ). Unexpectedly, after only 2–3 days (equivalent to 2–3 transfers or 7–10 generations) we observed a gradually increasing swimming polarity, with cells predominantly (>80%) accumulating at either the northern- or southernmost edge of the drop (SS or NS), depending on the direction of B during selection ( Fig. 5 ). Selected cells ( pol + ) were identical to non-selected cells ( pol − ) with respect to morphology, flagellation and appearance of the magnetosome chains. In contrast to non-selected cells that formed two similar aerotactic bands at each end of a flat capillary oriented parallel to B , selected cells formed a very dense band close to the meniscus at one end of the capillary and a fainter band more distant to the meniscus at the opposite end. Intriguingly, Δ cheOp1 cells lacked any swimming polarity, whether or not they had been grown under selective conditions, and accumulated in equal numbers at both edges of the hanging drop much like non-selected WT cells, suggesting oxygen and/or cheOp1 has a role in polarizing the magnetotactic response. To further study the influence of oxygen levels on the observed swimming polarity behaviour, we next analysed non-selected and NS WT cells in magnetic fields under defined conditions in a gas perfusion chamber. To measure the polarity bias at the single-cell level, we manually tracked the movements of individuals under anoxic conditions. As a measure for the relative polarity bias of individuals (PB ind ) we calculated the ratio of the relative time periods spent swimming either parallel or anti-parallel to B within 1-min intervals ( Supplementary Fig. 5 ). Resulting values between 0 and 0.5 reflected an overall directional bias of 50 to 100% towards the magnetic north pole, whereas values between 0 and −0.5 reflected a bias of 50 to 100% towards the magnetic south pole. While PB ind values of non-selected cells were widely scattered with an average of 0.04±0.27, those of NS cells ranged between −0.05 and 0.45 with an average of 0.17±0.17. This means that under anoxic conditions NS cells would gradually swim towards more oxic regions in an environment with the same oxygen gradient configuration as during NS polarity selection (north pole corresponds to high oxygen). To quantitatively estimate the polarity bias of entire populations, we video-tracked numerous swimming cells (in total ≧ 800) for a short time until they left the microscopic viewing field. From the distances covered by individuals both parallel and antiparallel to B we then calculated the mean polarity bias of the population (PB pop ). Under anoxic conditions, populations of NS cells displayed a slight but significant bias to swim anti-parallel to the magnetic field lines (PB pop =0.07, which means an idealized cell representing the whole population swam 57% towards the north pole and 43% towards the south pole) ( Supplementary Fig. 5b ). In contrast, consistent with ‘axial’ behaviour about equal portions of non-selected WT cells swam parallel or anti-parallel along B (PB pop =0.00). To further investigate the observed link between swimming polarity and aerotaxis, we analysed the response of polarity-selected cells to oxygen up-shifts, which we had found to cause a drastic temporary increase in reversal rates in non-magnetic cells. To this end, we modified the classical oxic hanging drop assay by placing microdroplets (1 μl) of selected WT cells in the gas perfusion chamber. Under anoxic conditions, most cells of a NS culture swam anti-parallel to B and accumulated at the northern edge of the drop ( Fig. 6a ). However, when the chamber was abruptly ventilated with 2% oxygen, within 2 s post-shift virtually all cells displayed multiple reversals that were followed by straight, long and uninterrupted runs parallel to B ( Supplementary Movie 6 ). Strikingly, this caused nearly the entire population to move uniformly towards the south pole. The overall directional change was due to swimming reversals parallel to field lines and not to cells performing U-turns, which are observed on reversal of B [29] . About 50% of the population had collectively left the northern edge 7 s post-shift, and within 90 s the vast majority of cells (we estimate >80%) had crossed the entire diametre of the drop (1–2 mm) and was accumulated at the opposite southern edge. Manual tracking of individuals before and after oxygen upshifts revealed that non-selected cells showed a very heterogeneous swimming pattern under both conditions ( Fig. 6b ). Many individuals lacked a clear behavioural response to the shift and did not reverse their swimming bias (as indicated by a change of sign of their PB ind ). The average PB ind therefore was close to zero under both conditions, which was corroborated by similar PB pop values obtained through automated mass tracking ( Fig. 6c , Supplementary Movie 8 ). This indicates that the ability to adjust the effective direction of movement after oxygen exposure is compromised in non-selected cells. In contrast, polarity-selected cells displayed a very uniform pattern. After the upshift PB ind values of NS cells on average decreased by 0.49 (compared with a mean absolute change of 0.19 in non-selected cells) and the majority of individuals reversed its swimming bias ( Fig. 6b ). Again, average PB ind values of selected cells were consistent with PB pop values in population tracking experiments that rapidly decreased from slightly positive to values around −0.3 after the shift and remained on a low level for >60 s ( Fig. 6c , Supplementary Movie 7 ). Analysis of individual cells for extended time periods post-shift further highlighted the described differences between selected and non-selected cells ( Supplementary Fig. 5d,f ). Last, equal numbers of cells swimming into either direction were observed for populations of Δ cheOp1 ( Supplementary Movie 5 ) and corresponding PB pop values were comparable to those of non-selected cells. 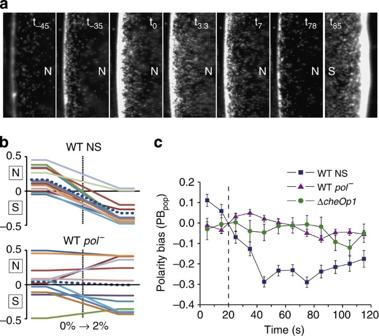Figure 6: Magnetic swimming polarity is switched by aerotaxis. (a) Dark field video recording ( × 100 magnification) of a reversing NS WT population in the gas perfusion chamber. Details of individual frames showing the edge of a drop corresponding to the north (N) or south pole (S). A 1-μl sample was equilibrated at 0% O2for 3 min before the recording was started. At t−40the sample was exposed to the magnetic field of a bar magnet. Time points of selected images (in s) are given in each image relative to an atmospheric shift from 0 to 2% O2(at t0). (b) Polarity bias of individual cells (PBind) calculated from swimming phase ratios as revealed by manual long-term tracking. Representative PBindplots of single NS (left,n=13)) and non-selected (pol−) WT cells (right,n=12) are shown. PBindvalues were calculated from 60-s intervals before and after a shift from 0 to 2% O2. Corresponding swimming directions relative to the magnetic field are given by N (anti-parallel) and S (parallel). The dotted blue line represents the mean of all analysed cells. (c) Polarity bias of populations (PBpop) that were shifted from 0 to 2% O2(indicated by dashed line) as revealed by automated mass tracking. The mean±s.e.m. of all individual cell bias values of selected (NS) WT, non-selected (pol−) WT and ΔcheOp1mutant cells are shown. For each graph data from 4 to 6 independent experiments were collected. Figure 6: Magnetic swimming polarity is switched by aerotaxis. ( a ) Dark field video recording ( × 100 magnification) of a reversing NS WT population in the gas perfusion chamber. Details of individual frames showing the edge of a drop corresponding to the north (N) or south pole (S). A 1-μl sample was equilibrated at 0% O 2 for 3 min before the recording was started. At t −40 the sample was exposed to the magnetic field of a bar magnet. Time points of selected images (in s) are given in each image relative to an atmospheric shift from 0 to 2% O 2 (at t 0 ). ( b ) Polarity bias of individual cells (PB ind ) calculated from swimming phase ratios as revealed by manual long-term tracking. Representative PB ind plots of single NS (left, n =13)) and non-selected ( pol − ) WT cells (right, n =12) are shown. PB ind values were calculated from 60-s intervals before and after a shift from 0 to 2% O 2 . Corresponding swimming directions relative to the magnetic field are given by N (anti-parallel) and S (parallel). The dotted blue line represents the mean of all analysed cells. ( c ) Polarity bias of populations (PB pop ) that were shifted from 0 to 2% O 2 (indicated by dashed line) as revealed by automated mass tracking. The mean±s.e.m. of all individual cell bias values of selected (NS) WT, non-selected ( pol − ) WT and Δ cheOp1 mutant cells are shown. For each graph data from 4 to 6 independent experiments were collected. Full size image Magnetosome-based magnetic navigation was discovered in bacteria almost 40 years ago [30] and has been implicated in the magnetoreception of higher organisms [31] , [32] . Since then various applications of bacterial magnetotaxis have been suggested, such as the transport of drugs or other cargo by magnetically steered bacterial microrobots in microfluidic systems or even blood vessels [33] , [34] . However, the biological mechanisms governing this behaviour and its integration with other sensory responses have remained unknown. Here, we demonstrate that polar magnetotaxis could be restored in the hitherto non-polar lab strain of M. gryphiswaldense, and this behaviour is tightly coupled with aerotaxis towards low-oxygen levels, the dominant chemotactic response of the bacterium. Chemotactic signal transduction in all bacteria is based on two-component systems involving autophosphorylation of the histidine kinase, CheA, followed by subsequent phosphotransfer to a response regulator, CheY [20] . We found that of the four identified chemotaxis operons of M. gryphiswaldense , only cheOp1 , comprising the canonical set of chemotaxis genes ( cheAWYBR ), is involved in aerotaxis and swimming polarity ( Fig. 7 ). cheOp1 encodes a hybrid CheA kinase and no CheZ, suggesting signal termination is through a phosphate sink, as in S. meliloti [35] . Owing to the absence of an MCP gene in cheOp1 and the great number of putative MCP-encoding genes ( Supplementary Table 3 ), an energy/oxygen sensor in M. gryphiswaldense has not been identified. In addition, the role of cheOp2-4 still remains unclear as the triple mutant lacked an obvious phenotype. This finding might suggest that, as in other bacterial species encoding multiple putative chemosensory pathways, these additional pathways may be controlling traits other than swimming behaviour [36] , which is supported by the identification of cyclic di-GMP-related motifs in cheOp2-4 . 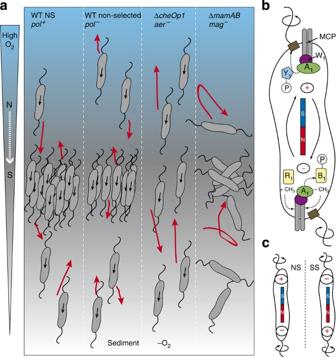Figure 7: Behavioural and molecular mechanism of polar magnetotaxis. (a) Schematic representation of polar magnetotaxis in magnetospirilla compared with the behaviour of mutants analysed in the study. Representative, idealized swimming tracks of individual cells in a vertical O2gradient aligned to the magnetic field (B) are shown as red arrows. Polar magnetotactic NS WT cells (pol+) form an aerotactic band at the oxic–anoxic transition (OAT). When displaced to hyper- or hypooxic zones, those cells avoid excursions into the ‘ecologically wrong’ direction and directly swim back to the OAT. In contrast, non-selected WT cells (pol−) swim in either direction relative toBand therefore their return to the OAT is slowed down. ΔcheOp1(aer−) mutant cells swim aligned toB, but fail to reverse and accumulate at favourable O2levels, while ΔmamAB(mag−) mutant cells behave similar to other non-magnetotactic bacteria and only use temporal gradient sensing to steer towards the OAT. (b) Molecular components underlying aerotaxis and swimming polarity in magnetospirilla. CheA, CheW, CheY, CheB and CheR of CheOp1 are shown (CheY1, CheB1and CheR1depicted only at one pole to avoid crowding). The histidine kinase CheA1phosphorylates CheY1, which in its activated form binds to the motor complex causing motor reversals. Direction of flagella rotation is indicated by circular arrows, the bar magnet indicates magnetic (M) polarity. A hypothetical polarity marker (reflecting cellular (C) polarity) gradually influencing motor output is marked with +/− symbols. (c) Hypothetical C polarity of NS and SS cells (indicated by +/− axis) resulting in opposite motor output (indicated by arrows). Figure 7: Behavioural and molecular mechanism of polar magnetotaxis. ( a ) Schematic representation of polar magnetotaxis in magnetospirilla compared with the behaviour of mutants analysed in the study. Representative, idealized swimming tracks of individual cells in a vertical O 2 gradient aligned to the magnetic field ( B ) are shown as red arrows. Polar magnetotactic NS WT cells ( pol + ) form an aerotactic band at the oxic–anoxic transition (OAT). When displaced to hyper- or hypooxic zones, those cells avoid excursions into the ‘ecologically wrong’ direction and directly swim back to the OAT. In contrast, non-selected WT cells ( pol − ) swim in either direction relative to B and therefore their return to the OAT is slowed down. Δ cheOp1 ( aer − ) mutant cells swim aligned to B , but fail to reverse and accumulate at favourable O 2 levels, while Δ mamAB ( mag − ) mutant cells behave similar to other non-magnetotactic bacteria and only use temporal gradient sensing to steer towards the OAT. ( b ) Molecular components underlying aerotaxis and swimming polarity in magnetospirilla. CheA, CheW, CheY, CheB and CheR of CheOp1 are shown (CheY 1 , CheB 1 and CheR 1 depicted only at one pole to avoid crowding). The histidine kinase CheA 1 phosphorylates CheY 1 , which in its activated form binds to the motor complex causing motor reversals. Direction of flagella rotation is indicated by circular arrows, the bar magnet indicates magnetic (M) polarity. A hypothetical polarity marker (reflecting cellular (C) polarity) gradually influencing motor output is marked with +/− symbols. ( c ) Hypothetical C polarity of NS and SS cells (indicated by +/− axis) resulting in opposite motor output (indicated by arrows). Full size image Bacterial taxis in chemical gradients is generally accomplished by a combination of straight-line swimming and reversing or reorienting. As has been shown for other polarly flagellated bacteria [37] , [38] , M. gryphiswaldense does not tumble between smooth swimming phases, but instead swims in a typical run and reversal pattern, with speeds between 20 and 65 μm s −1 , similar to previously reported values [12] , [13] , [39] . In equilibrium conditions, cells showed a reversal frequency of 0.126 s −1 or less, which is low compared with data reported for non-MTB [40] , [41] , [42] , [43] . Consistent with the adaptation of MTB for growth in redox gradients in stratified sediments [27] , and also with the dependence of oxygen-sensitive magnetite biomineralization and N 2 fixation on suboxic conditions [44] , [45] , we found a higher proportion of cells swam faster and reversed less frequently under microoxic than under anoxic or fully oxic conditions. The model of energy taxis suggests cells swimming towards lower or higher oxygen concentrations would experience a change in proton motive force or electron transfer rates [15] , [46] , resulting in increased motor reversals. However, on temporal oxygen-upshifts, M. gryphiswaldense displayed a very different behavioural response: a short period of highly increased reversal frequency was followed by a rapid and prolonged decrease of reversals, resulting in straight, uninterrupted runs, very different from the prestimulus state. This is in contrast to other bacteria, which typically display a return to prestimulus levels after responding to repellent stimuli [46] , mediated through adaptation and resetting of the receptor proteins. The presence of genes encoding conserved adaptation proteins, CheB and CheR, in cheOp1 suggests that adaptation occurs, but also implies that adaptation resets the CheA signalling state to one tuned to the new environment. This distinct behavioural pattern of M. gryphiswaldense resembling a form of ‘escape response’ would rapidly guide the cells back to suboxic environments after displacement into hyperoxic, harmful zones ( Fig. 7 ) and would prove beneficial in environmental redox gradients, which are prone to strong temporal and spatial changes. Aerotactic signalling through CheOp1 was essential for magnetic swimming polarity. Contrary to the prevailing model, we show that instead of using the magnetic field only as an axis, M. gryphiswaldense is capable of polar magnetotaxis. Swimming polarity appeared to be an inherent property of cells, and the temporary loss of motility bias after non-selective lab cultivation was not caused by genetic loss, but could be restored by appropriate incubation within oxygen gradients superimposed with magnetic fields mimicking the geomagnetic inclination. As all MTB including magnetospirilla sampled from environmental sites generally display swimming polarity [3] , [26] , [27] , it seems likely that in natural redox gradients in which cells persistently experience polarity selection by the geomagnetic field vector polar rather than ‘axial’ magnetotaxis is the prevalent mode of magnetic navigation common to all MTB. The previously observed ‘axial’ behaviour of magnetospirilla therefore might represent an artefact, resulting from the loss of selection during lab cultivation. Selection is probably explained by the cells with the appropriate bias being directed more efficiently towards favourable growth conditions, gradually outcompeting others more regularly exposed to more harmful oxygen concentrations. Selection of swimming polarity was not caused by enrichment of pre-existing unidirectional NS or SS bacteria equally prevalent in non-selected populations, but instead resulted from a gradually increased bias at the single-cell level by which one swimming direction became favoured over time ( Fig. 6b and Supplementary Fig. 5 ). In addition, non-selected cells failed to display a clear switch of swimming bias on oxic shifts, although overall reversal rates were not affected. Thus, the propensity of individual cells to respond towards one particular direction under anoxic conditions and to reverse the effective direction in the presence of high oxygen was gradually selected. Increasing run lengths when swimming with one cellular pole ahead is in contrast to other bacteria that exhibit no intrinsic polarity in swimming behaviour. For instance, the sensory system of E. coli does not favour one swimming direction over the other [47] . Directional motility requires a fixed orientation of the in-build magnetic moment (M polarity) with respect to the sense of flagellar rotation (reflecting C polarity). It has proved impossible so far to directly visualize the rotation of individual filaments, but for directional motility both motors would turn with opposite senses of rotation, and motor reversals have to be coordinated between the opposing poles (resulting in switching between leading and trailing flagella). This simultaneous motor activity has been observed in other spirilla with bipolar flagellation [37] , [48] and is also consistent with our observations on tethered cells, which never displayed extended stops as would be expected if the motors rotated and paused alternately. However, the sense of flagellar rotation also depends on the concentration of CheY~P. It seems improbable that the cell establishes a gradient of CheY~P between the two cell poles that is instantaneously reversed during swimming reversals. In addition, due to the small size of the bacterial cell the chemotaxis receptors at both poles sense the same stimulus, which probably leads to the same CheY phosphorylation level at both poles. Therefore, the direction of motor rotation might be ‘hardwired’ into each motor, so that at a low CheY phosphorylation level one motor turns CW while the other turns CCW, and vice versa at higher phosphorylation levels. At the moment, it is unclear how swimming polarity is determined at the cellular and molecular level. We failed to detect any polarity selection or a reversible swimming bias in cells lacking cheOp1 . This highlights that magnetic swimming polarity depends on signalling via CheOp1 and is not autonomously controlled by a dedicated sensory pathway exclusively serving magnetotaxis. However, the observed behaviour cannot be fully explained by a simple temporal sensing mechanism, as in this case cells would be expected to exhibit equally timed average swim phases with each pole ahead. As already noted by Frankel et al. [6] , polar magnetotaxis might involve a means to measure absolute oxygen concentrations. Unlike magnetic cocci, which have inherent C polarity owing to their asymmetric monopolar flagellation ( Supplementary Fig. 5h ), bipolarly flagellated spirilla exhibit apparently symmetric morphology. So far, we can also only speculate about what determines the C polarity axis in magnetospirilla, but it is clear that the relative output of the motors of NS and SS cells has to be opposite, and, therefore, swimming polarity must be based on some sort of symmetry breaking at subcellular level (C polarity symbolized by ‘+’ and ‘−’ in Fig. 7 ) parallel to the M polarity axis. As CheW 1 -GFP fusions show a bipolar localization pattern in both polarity-selected and non-selected cells similar as observed in other magnetospirilla [49] , asymmetric chemoreceptor localization, however, appears to be an improbable mechanism. For instance, a spatial bias might be established by a modification of motor components, an uneven distribution of signal transduction components or of a dedicated marker molecule. There are precedents for C polarity-determining factors and plasticity of polar identity in other bacteria [50] , even though the molecular processes controlling polarity axis redefinition are largely unknown. It had been proposed by Lumsden that after cell division swimming polarity might be inherited non-genetically by daughter cells via the M polarity of the inherited magnetosome chain [51] . However, swimming polarity was selected in M. gryphiswaldense within fewer than 10 generations, suggesting that selection is independent of the rarely occurring loss through missegregation and de novo formation of the magnetosome chain. Our data also argue against a rapid, merely physical effect of re-magnetization (reversal of M polarity) caused by exposure to artificial magnetic fields, but point to a mechanism that gradually defines, modifies and passes on the relative orientation of the magnetotactic C polarity axis of magnetospirilla. In conclusion, we demonstrate that polar magnetotaxis can be selected even in magnetospirilla thus far believed to be non-polar, and this magnetic swimming polarity is controlled by aerotactic signal transduction through CheOp1. Contrary to previous assumptions that magnetotaxis is passive and independent of sensory pathways, we provide first evidence for a genetic link between aero- and magnetotaxis and magnetotactic polarity. Bacterial strains, plasmids and culture conditions Bacterial strains and plasmids used in this study are listed in Supplementary Tables 4 and 5 . For genetic experiments M. gryphiswaldense strains were grown microaerobically in modified flask standard medium (FSM) at 30 °C under moderate agitation (120 r.p.m.) [45] . To grow E. coli BW29427, 1 mM DL-α, ε-diaminopimelic acid (DAP) was added to LB medium. For strains carrying recombinant plasmids, media were supplemented with 25 g ml −1 kanamycin, 12 g ml −1 tetracycline and 15 g ml −1 gentamicin for E. coli strains, and 5 g ml −1 kanamycin, 5 g ml −1 tetracycline and 20 g ml −1 gentamycin for M. gryphiswaldense strains, respectively. Molecular and genetic techniques The draft genome sequence of M. gryphiswaldense (GenBank accession number CU459003) was used for primer design. Oligonucleotides were purchased from Sigma-Aldrich (Steinheim, Germany). All constructs were sequenced on an ABI 3700 capillary sequencer (Applied Biosystems, Darmstadt, Germany), utilizing BigDye Terminator v3.1. Sequence data were analysed with Geneious Software (Biomatters). Using both E. coli CheA and R. sphaeroides CheA2 sequences as a query in BlastP searches, we identified four predicted proteins with strong similarity (E-value below E−40) that were encoded on several contigs of the draft genome sequence of M. gryphiswaldense . Genes neighbouring the four cheA sequences were identified by alignment with the known sequences of M. magneticum AMB-1, M. magnetotacticum MS-1 and M. marinus MC-1 on nine different contigs in the M. gryphiswaldense genomic assembly. Gaps between contigs were closed by bridging PCR reactions ( Supplementary Table 5 ) resulting in four contiguous operon sequences ( Supplementary Table 2 ). Plasmids were constructed by standard recombinant techniques. For deletion mutagenesis upstream and downstream fragments of all operons were amplified by PCR with primers including suitable restriction sites ( Supplementary Table 5 ) and ligated into pAL01_MCS1 and pAL02/2_MCS2, respectively, resulting in pFP01 and pFP04 to pFP10. Deletion mutant strains were obtained by a two-step conjugation method involving cre-lox recombination as described before [24] . Resulting mutant strains ( Supplementary Table 4 ) were verified by PCR reactions with primers binding to genomic sequences outside of the homologous regions used for plasmid integration ( Supplementary Table 5 ). Successful deletions were checked by sequencing the obtained PCR products. For the complementation of strain FP20 (MSR Δ cheOp1 ), the cheOp1 sequence was amplified from genetic DNA with primers fp13 and fp71 and subcloned into pJet1.2. After digestion the fragment was ligated into pOR093 to obtain pFP11. This plasmid was used to obtain strain FP56 through a two-step homologous recombination method using galK -based counterselection [52] . Culture conditions for motility experiments After testing of different cultivation parameters (inoculum size, cultivation temperature, oxygen concentration, medium composition and incubation time) we found that, using a small inoculum (OD 0.005), preculturing the cells under denitrifying conditions, as well as harvesting young, early logarithmic phase cells (OD 0.05), yielded maximum motility. Therefore, cells were grown under these conditions and diluted in FSM medium where needed in all subsequent chemotaxis experiments. For selection of polarity, cells were cultured in Hungate tubes that had been sparged with 98% N 2 /2% O 2 mixtures before autoclaving. Hungate tubes were placed in a Helmholtz coil cage ( Supplementary Fig. 4a ) and subjected to vertical magnetic fields of 0.57 mT (~10 × the geomagnetic field strength) during growth for at least two serial transfers. Magnetic fields were applied either parallel (north pole→south pole) or antiparallel (south pole←north pole) to oxygen gradients in the tubes (Ox Low →Ox High ). For release of magnetic selection Hungate tubes were agitated on a tube rotator at 60 r.p.m. Chemotaxis experiments To test for tactic reactions, we performed a set of classical chemotaxis experiments (swarm plates [8] , plug-in-pond assays [53] , mini-plug slides [54] , commercial microscope slide chemotaxis chambers (μ-slide chemotaxis, Ibidi GmbH [16] ) with different carbon sources as putative attractants (lactate, pyruvate, acetate). Swarming occurred in soft agar with all chemicals tested, but no positive responses were detected in any other assay performed. Also light of different wavelengths did not have a detectable effect. In mini-plug assays band formation was observed even in the absence of any chemical in the plug. This pointed towards a strong aerotaxis response that possibly overrides other tactic reactions. For the preparation of gradient soft agar tubes the FSM medium was modified by supplementing 0.3% agar, adding only 1.5 mM lactate (10% of normal concentration) and omitting peptone and nitrate. A 10 ml of sterile soft agar was poured into test tubes, and 100 μl of a microoxically grown overnight culture was dispersed into the agar. Tubes were incubated at 30 °C under oxic conditions for 2 days. To test taxis towards nitrate, a vertical nitrate gradient was preformed in anoxic soft agar tubes by an agar plug at the bottom of test tubes containing variable nitrate concentrations (0, 10 and 100 mM). A 50 ml of an overnight batch culture was washed once in nitrate-free 10 mM HEPES buffer pH 7, resuspended in 500 μl buffer, mixed with 0.3% nitrate-free soft agar and directly poured onto previously prepared agar plugs. Tubes were directly transferred to an anaerobic glove box and incubated for 4 h. Nitrate concentration at the position where the band had formed was analysed by taking agar samples with a Pasteur pipette and using a commercial Szechrome reagent nitrate quantification kit (Polysciences). For the preparation of swim plates only 0.2% agar was used, the concentration of carbon source (lactate) was lowered to 1.5 mM and peptone was omitted from FSM medium. Five microlitres of overnight culture was pipetted into the swim agar and plates were incubated under microxic conditions for 2 days (protocol modified from ref. 8 ). Video microscopy and analysis of swimming parameters Swimming behaviour of cells was analysed and recorded using dark-field microscopy on an upright Zeiss Axioplan microscope (Zeiss, Jena, Germany) at × 100 magnification. Cells tethered spontaneously to the coverslip by one of their flagella were recorded at × 400 magnification and 43 fps. For routine observation of swimming populations, 5 μl of an OD 0.1 cell suspension was placed under a coverslip and sealed with nail varnish. For aerobic hanging drop assays, 3 μl of cell suspension was pipetted onto a coverslip that was placed upside-down on an O-ring ( Supplementary Fig. 4b ). All other motility experiments were performed within a microscopic gas perfusion chamber (Ludin Chamber, Life Imaging Services) that was equilibrated with variable moisturized and precisely adjusted O 2 -N 2 gas mixtures containing between 0 and 21% oxygen ( Supplementary Fig. 2 ). As the quantititative analysis of freely swimming WT cells was hampered by their tendency to align magnetically and distribute inhomogenously within the sample droplets, basic swimming characteristics in equilibrium conditions were analysed in the non-magnetic Δ mamAB strain. Homogeneous conditions within sample droplets were maintained by using strongly diluted cell suspensions (OD 0.005) and placing 0.25 μl droplets of cell suspension under a constant gas flow of 50 ml min −1 . Videos were recorded with a UK1158–M camera (EHD, Damme, Germany) at a frame rate of 15 fps and a standard resolution of 1360 × 1024 pixels using VirtualDub software. Dark-field video records were analysed by a custom-made automated tracking software (‘WimTaxis—Bacteria Tracking’, Wimasis GmbH, München, Germany) specifically adapted to determine basic swimming characteristics. The software automatically detected swimming reversals and provided the x - y coordinates of every tracked cell for each frame. The minimum track length was set to be 50 frames. Within the usual tracking times (depending on the time bacteria stayed in the viewing field, usually below 10 s) reversals generally were too infrequent to simply average reversal rates of single cells. Therefore, the reversal frequency analysis for each experiment was performed at the population level, and all detected reversals were divided by the total respective tracking time (sum of the temporal length of all tracks) to obtain the population average. For the analysis of switching behaviour at different equilibrium oxygen levels, reversal frequencies were determined for each video, and the mean and s.d. of five to nine such independent experiments were determined. To illustrate the biological variability of swimming speed, the curvilinear speed values (track length divided by tracking time) corresponding to individual tracks from all independent experiments were pooled to calculate the average speed of all tracked cells. To analyse the cell reaction to oxygen shifts, the gas stream was manually switched between oxic and anoxic. For this purpose we equipped our set-up with a three-way valve and a flow meter to adjust the flow of N 2 gas to 50 ml min −1 ( Supplementary Fig. 2a ). To determine the average reversal frequency over time, the number of detected reversals within 5-s intervals was added up from three independent video recordings and normalized to the total corresponding tracking time. To calculate mean speeds within the same 5-s intervals the instantaneous speeds (derived from the increment in x and y per frame per cell) of all tracks extending into the same window were averaged. Analysis of swimming polarity To analyse swimming polarity we used a modified version of the magnetodrome [55] to create homogenous tunable magnetic fields parallel to the focal plane of our microscope ( Supplementary Fig. 2a ). Magnetodrome software was used to control two pairs of coils in Helmholtz configuration, and a field strength of 0.26 mT (parallel to the y -axis of the viewing field) was used in all polarity experiments. The behaviour of polarity-selected populations was assayed by placing 0.25 μl sample droplets onto the lower coverslip of the gas perfusion chamber. After equilibration with N 2 gas for 3 min the magnetic field was switched on. After 40 s the atmosphere was shifted to 2% O 2 and the behaviour of the population was recorded. To determine the polarity bias of individual cells, the number of focal planes within the liquid phase had to be minimized. For this purpose 1 μl of sample was sandwiched between the coverslip of the perfusion chamber and a thin agar slice. The movements of individual cells were followed manually and video-recorded. From the cumulated time periods swimming either parallel (t south ) or anti-parallel to B (t north ) within 1-min intervals, the population bias of individual cells (PB ind ) was calculated: When cells were tracked for extended time periods ( Supplementary Fig. 5d ,f), PB ind was calculated from all available data. To quantitatively estimate the polarity bias of populations, we recorded 3–6 videos (40 s each for equilibrium conditions, 120 s each for shift experiments), and all swimming cells within the viewing field were tracked automatically. From the cumulated swimming distances of single cells within 10-s intervals, either anti-parallel to B (d north ) or parallel to B (d south ), the polarity bias of individuals (PB distance ) was calculated. The mean polarity bias of the population (PB pop ) over time was obtained by averaging the bias values of all individually tracked cells within the same intervals. How to cite this article: Popp, F. et al. Polarity of bacterial magnetotaxis is controlled by aerotaxis through a common sensory pathway. Nat. Commun. 5:5398 doi: 10.1038/ncomms6398 (2014).